Engineered microbial biofuel production and recovery under supercritical carbon dioxide Culture contamination, end-product toxicity, and energy efficient product recovery are long-standing bioprocess challenges. To solve these problems, we propose a high-pressure fermentation strategy, coupled with in situ extraction using the abundant and renewable solvent supercritical carbon dioxide (scCO 2 ), which is also known for its broad microbial lethality. Towards this goal, we report the domestication and engineering of a scCO 2 -tolerant strain of Bacillus megaterium , previously isolated from formation waters from the McElmo Dome CO 2 field, to produce branched alcohols that have potential use as biofuels. After establishing induced-expression under scCO 2 , isobutanol production from 2-ketoisovalerate is observed with greater than 40% yield with co-produced isopentanol. Finally, we present a process model to compare the energy required for our process to other in situ extraction methods, such as gas stripping, finding scCO 2 extraction to be potentially competitive, if not superior. Supercritical fluids offer many advantages over conventional solvents due to their gas-like viscosity and diffusivity with liquid-like density and solvation [1] . Supercritical carbon dioxide (scCO 2 ) is especially promising as a green solvent due to its moderate critical point temperature (31.1 °C) and pressure (7.38 MPa) as well as being non-flammable, non-hazardous, abundant, and inexpensive [2] . Numerous biocatalytic processes have taken advantage of scCO 2 [2] , [3] , including enantiomer specific lipase reactions [4] , asymmetric alcohol reduction [5] , and carboxylation of various substrates [6] . The solvent properties of scCO 2 have been exploited for the separation of alcohols, aldehydes, ketones, and acids from aqueous solutions via both in situ and ex situ extraction [7] . In situ product extraction has been shown to have a dramatic effect on bioproduction titers by alleviating end-product inhibition or toxicity [8] , [9] , [10] , [11] . scCO 2 is especially attractive within biphasic scCO 2 -aqueous systems [12] due to its preferential extraction of alcohols with intermediate-chain length (e.g., 3 to 6 carbons), the result of decreasing water solubility with increasing number of carbons. Conversely, alcohol volatility decreases with chain length, making these molecules more attractive targets for scCO 2 extraction compared to gas stripping [12] . Despite the potential to couple scCO 2 for product removal with microbial synthesis of target compounds, the two have not been combined due to the broad microbial lethality of scCO 2 [13] , where cellular inactivation is thought to occur through a combination of membrane disruption, cytosolic acidification, enzyme inactivation, and cellular desiccation [14] . Several early studies have explored processes catalyzed by whole cells under scCO 2 ; however, these were conducted over short time scales ( < 1 day) using biomass grown in the absence of scCO 2 , and without evidence of cell viability under scCO 2 . Two results include carboxylation of pyrrole substrate with Bacillus megaterium cells in a biphasic mixture of buffered solution and scCO 2 after 1 h [15] , and reduction of ketones with a high degree of enantiomer specificity using immobilized Geotrichum candidum cells in an aqueous-scCO 2 biphasic continuous flow reactor [16] . Several additional studies have employed scCO 2 -based extraction of bioproducts, but have not achieved in situ extraction due to inhibited cell growth. Using a semi-continuous process, ethanol was extracted from the spent fermentation broth of yeast [17] and Clostridium [18] cultures using scCO 2 . Knutsen et al. [19] attempted to produce ethanol from cellobiose in dual-phase aqueous bioreactors containing non-growing Clostridium thermocellum and pressurized scCO 2 , N 2 or ethane headspaces. Significant cellobiose conversion and ethanol production were observed under pressurized nitrogen and ethane, but not under scCO 2 [19] , indicating process inhibition by CO 2 . Bioprospecting is a promising approach to recover organisms capable of active metabolism under high pressures of CO 2 . Numerous environmental isolates have been characterized with tolerance to high partial pressures of CO 2 [20] , although rarely are cultures examined above atmospheric pressures (0.1 MPa). Santillan et al. [21] found a strain of Lactobacillus casei in a terrestrial CO 2 -rich spring that can grow in CO 2 pressures up to 1 MPa. Recently, Peet et al. [22] examined organisms capable of growth at geologic CO 2 sequestration sites, isolating several endospore-forming Bacillus species that are tolerant to scCO 2 treatment ( > 10 MPa), but with low growth frequency and magnitude. Similarly, growth was reported for laboratory cultures inoculated with deep subsurface sandstone under scCO 2 , although the identities of microorganisms were not determined [23] . Motivated by the hypothesis that natural deposits of high-pressure CO 2 would harbor microorganisms adapted to actively grow in close contact with it, Freedman et al. [24] investigated the microbial diversity at McElmo Dome, a deep subsurface CO 2 reservoir that was formed 40–72 million years ago. Laboratory enrichment cultivation of fluids collected from McElmo dome under scCO 2 enabled isolation of B. megaterium strain SR7, an endospore-forming, facultative-anaerobe [25] . We have observed growth of SR7 cultures to a cell density of greater than 10 7 cells ml –1 after 3 weeks under scCO 2 following inoculation as endospores and supplementation with the germination inducer l -alanine [25] . Endospores of Gram-positive bacteria are known for their resiliency even when exposed directly to scCO 2 [22] , [26] , and we have hypothesized that this dormant state enables these bacteria to withstand and adapt to the scCO 2 environment prior to outgrowth as vegetative cells. Analysis of fermentation products from SR7 grown under scCO 2 indicated the production of lactate, acetate and succinate, demonstrating active metabolism under scCO 2 and the potential for microbial production to be coupled with scCO 2 extraction [25] . In this work, we seek to develop B. megaterium SR7 as a bioproduction host under scCO 2 for useful compounds that have already been established for in situ extraction using scCO 2 (Fig. 1 ), such as branched, intermediate-chain alcohols. We posit that an integrated fermentation-scCO 2 extraction process may ultimately, and simultaneously, solve three long-standing challenges in the field by (1) reducing end-product toxicity through extraction [9] , [10] , [11] , (2) mitigating culture contamination under the highly selective conditions of scCO 2 [13] , [22] , [25] , and (3) providing an energy efficient method to recover high-purity products using scCO 2 as a sustainable solvent [1] , [12] . Branched, intermediate-chain alcohols are not naturally made by SR7, necessitating metabolic engineering to generate them [25] . Isobutanol is selected due to its importance as a drop-in replacement for gasoline and its favorable fuel characteristics (i.e., high energy density, suitable research octane number, low hygroscopicity). Additionally, isobutanol is an attractive molecule for in situ scCO 2 extraction as it is cytotoxic and expected to partition favorably to the scCO 2 phase [7] , [12] . Isobutanol production requires introduction of two heterologous enzymes, an α-ketoisovalerate decarboxylase and alcohol dehydrogenase, to convert the valine-synthesis intermediate, 2-ketoisovalerate, to the final product with minimal intermediate isobutyraldehyde accumulation [27] . We conclude our study by analyzing the energy requirements of an integrated fermentation-extraction process, comparing it to alternative in situ extraction technologies such as gas stripping, pervaporation, and adsorption [28] , in order to address challenges associated with energy efficient product recovery. Fig. 1 Schematic of integrated fermentation and extraction under supercritical CO 2 . A scCO 2 -tolerant microbe can be engineered to produce compounds, such as medium-chain alcohols (C4-C5), that may serve as biofuels and may be preferentially extracted from aqueous media into the scCO 2 phase. Collection of scCO 2 followed by partial de-pressurization will facilitate high-purity biofuel extraction. The presented biphasic scCO 2 separation strategy is expected to simultaneously provide a contaminant-free environment for the engineered organism due to the broad microbial lethality of scCO 2 , and continuously strip microbially produced biofuels to eliminate end-product toxicity. scCO 2 is only weakly soluble in the aqueous media phase ( < 1%) and vice versa, resulting in a biphasic system Full size image Heterologous protein expression in aerobically grown SR7 As strain B. megaterium SR7 is an environmental isolate, its genetic modification required optimization and customization of protocols previously developed for laboratory strains and model organisms. A transformation protocol for SR7 was developed by modifying a method based on protoplast-osmotic shock [29] (Supplementary Note 1 ). The xylose-inducible promoter system (pXyl) was selected for use in SR7 due to its simplicity, high expression level, and widespread use in the B. megaterium literature [29] (Fig. 2a ). Additionally, the IPTG-inducible hyperspank promoter system (pHysp) [30] and the p43-growth based promoter (p43) were evaluated, both of which have shown effective protein production in B . subtilis [31] (Fig. 2a ). Fig. 2 Heterologous protein expression and promoter evaluation in SR7. a Schematic of the promoters tested in SR7. pXyl is a xylose-inducible promoter and contains the xylR gene and xylA promoter from B. megaterium strain DSM 319. pHysp contains the IPTG-inducible hyperspank promoter and lacI , both from plasmid pDR111. The p43 promoter is taken from B. subtilis strain KS438 and is growth-associated. Expected inducers are indicated in parentheses. b Bulk fluorescence measurements of SR7 populations containing gfp- encoding plasmids, with (circles, solid lines) or without (diamonds, dashed lines) inducers. Error bars represent the standard deviation of biological triplicate samples. c Fluorescence populations of SR7 cells expressing gfp at 4 h post induction measured by FACS (Alexa Fluor 488). A GFP positive gate was established using the autofluorescence of SR7 cells containing an empty plasmid control. d Phase-contrast and fluorescence microscopy of SR7 pXyl gfp cells with and without xylose induction. Images were taken 4 h post induction. Source data are provided as a Source Data file Full size image All three promoters were functional in SR7 (Fig. 2b and Supplementary Fig. 1 ), with pXyl and pHysp promoters resulting in strong GFP expression of 25- and 20-fold greater than uninduced cultures, respectively. The xylose promoter was activated most rapidly, achieving maximal fluorescence 3 h post induction, similar to other B. megaterium strains using this promoter system [32] . For induced pXyl gfp and pHysp gfp cultures, a large proportion ( > 95%) of the population was found to express GFP (Fig. 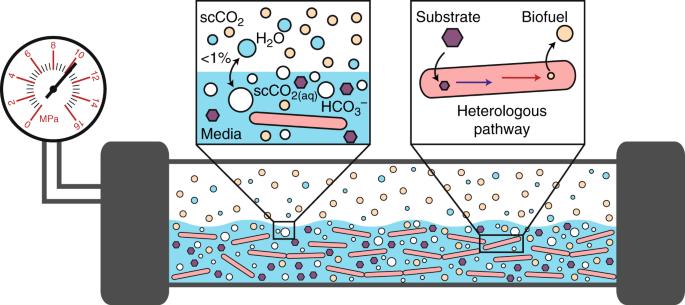Fig. 1 Schematic of integrated fermentation and extraction under supercritical CO2. A scCO2-tolerant microbe can be engineered to produce compounds, such as medium-chain alcohols (C4-C5), that may serve as biofuels and may be preferentially extracted from aqueous media into the scCO2phase. Collection of scCO2followed by partial de-pressurization will facilitate high-purity biofuel extraction. The presented biphasic scCO2separation strategy is expected to simultaneously provide a contaminant-free environment for the engineered organism due to the broad microbial lethality of scCO2, and continuously strip microbially produced biofuels to eliminate end-product toxicity. scCO2is only weakly soluble in the aqueous media phase ( < 1%) and vice versa, resulting in a biphasic system 2c, d and Supplementary Table 1 ), which is greater than that observed for other B. megaterium strains using pXyl [33] . Uninduced pXyl gfp containing cells have many members (40%) that fall into the GFP positive gate, providing evidence that this promoter is leaky when grown aerobically in rich Luria-Bertani (LB) medium (Supplementary Table 1 and Supplementary Fig. 2 ), in contrast to previous work showing tight regulation of pXyl within B. megaterium strain WH320 [32] . As expected, the growth-associated p43 promoter was activated as the cells entered exponential growth phase (Supplementary Fig. 1e, f ), but showed weaker GFP expression, only sixfold greater than the empty plasmid-containing control strain. Inducible production of GFP for the pXyl and pHysp promoters was also observed for cells cultured in semi-defined medium supplemented with xylose and/or glucose, with maximal fluorescence observed for cells containing the pXyl promoter grown in xylose-amended medium (Supplementary Fig. 3 ). Expression of gfp from the xylose promoter was shown to be lowered when both glucose and xylose sugars are present, likely due to catabolite repression, as observed for other strains of B. megaterium [34] , [35] (Supplementary Fig. 4 ). Based on the rapidity, strength, and uniformity of induction, the remaining work presented herein utilized the pXyl promoter. Plasmid retention was assessed, as the literature is mixed regarding long-term exogenous plasmid stability in B. megaterium [36] , [37] . 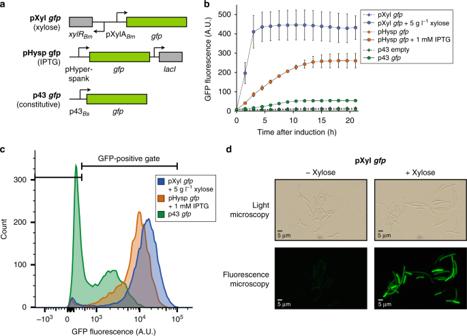Fig. 2 Heterologous protein expression and promoter evaluation in SR7.aSchematic of the promoters tested in SR7. pXyl is a xylose-inducible promoter and contains thexylRgene andxylApromoter fromB. megateriumstrain DSM 319. pHysp contains the IPTG-inducible hyperspank promoter andlacI, both from plasmid pDR111. The p43 promoter is taken fromB. subtilisstrain KS438 and is growth-associated. Expected inducers are indicated in parentheses.bBulk fluorescence measurements of SR7 populations containinggfp-encoding plasmids, with (circles, solid lines) or without (diamonds, dashed lines) inducers. Error bars represent the standard deviation of biological triplicate samples.cFluorescence populations of SR7 cells expressinggfpat 4 h post induction measured by FACS (Alexa Fluor 488). A GFP positive gate was established using the autofluorescence of SR7 cells containing an empty plasmid control.dPhase-contrast and fluorescence microscopy of SR7 pXylgfpcells with and without xylose induction. Images were taken 4 h post induction. Source data are provided as aSource Datafile Plasmid retention ( > 87%) was verified after 74 h of culturing by counting colony forming units (CFUs) on media with and without antibiotic selection as well as confirming the presence of plasmid elements for individual colonies (Supplementary Table 2 and Supplementary Fig. 5 ). Heterologous protein production in SR7 grown under scCO 2 The anaerobic functionality of the xylose promoter was next established for SR7 grown under 0.1 MPa CO 2 (i.e., atmospheric pressure) as well as a 10 MPa headspace of scCO 2 . Several challenges were anticipated when moving from aerobic to scCO 2 -based culturing, including slower and less predictable growth due to stresses associated with scCO 2 , and reduced maintenance of non-native plasmids through sporulation, germination, and outgrowth. Since the formation of the GFP chromophore is oxygen dependent, the β-galactosidase protein (LacZ) from E. coli was selected as a reporter for anaerobic cultures due to its previous use in B. megaterium [32] , its oxygen independence, and its easy and sensitive detection via enzymatic assay. After confirming heterologous lacZ expression (Fig. 3 ) and plasmid maintenance under 0.1 MPa CO 2 (Supplementary Note 2 ), the functionality of the pXyl promoter was assessed for SR7 pXyl lacZ cells grown under 10 MPa scCO 2 at 37 °C in semi-defined medium containing glucose as a carbon source and l -alanine as a germination inducer [25] . Xylose was added as an inducer at the time of inoculation rather than during early exponential growth since high-pressure cultivation of SR7 in stainless steel columns precludes non-destructive amending of samples during cultivation. After 21 days of incubation under scCO 2 , LacZ activity was measured in crude lysates derived from columns that displayed growth. Cells grown under 0.1 MPa and 10 MPa CO 2 with xylose displayed similar LacZ specific activities of 0.56 and 0.40 U mg –1 , respectively (Fig. 3 ). The 15-fold increase in LacZ expression under 10 MPa relative to uninduced cultures ( p = 0.0059) is similar in magnitude to the increase in induced-expression observed under 0.1 MPa (Fig. 3 ). Fig. 3 β-Galactosidase activity for SR7 cultures grown under 0.1 MPa CO 2 and 10 MPa scCO 2 at 37 °C. Specific β-galactosidase activity measured in lysates of SR7 cultures that contain an empty pXyl plasmid or pXyl lacZ . Activity was normalized to total protein concentration in the lysate to control for growth differences and differential cell lysis. Errors represent standard deviation of biological replicate cultures ( n > 4). For cultures grown under 0.1 MPa CO 2 , overnight anaerobic cultures grown from spores were subcultured into CO 2 -evacuated vials to a uniform optical density. Induction with xylose occurred 2 h after subculture, and the time point for LacZ activity measurement was taken 4 h post induction. For cultures grown under 10 MPa scCO 2 , SR7 pXyl lacZ spores were loaded into stainless steel culture vessels with and without xylose inducer. Cultures were grown for 21 days and microscopy was used to determine which samples showed at least a tenfold increase in cell number prior to measuring LacZ activity. Source data are provided as a Source Data file Full size image Growth of SR7 from endospores under scCO 2 has been defined as at least a tenfold increase in cell number and presence of vegetative cells, as determined by direct cell counts using fluorescence microscopy [25] . 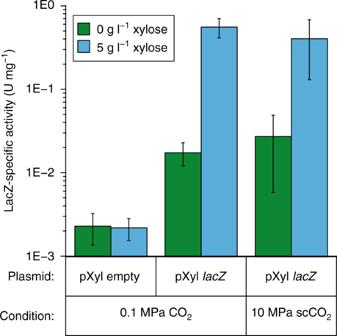Fig. 3 β-Galactosidase activity for SR7 cultures grown under 0.1 MPa CO2and 10 MPa scCO2at 37 °C. Specific β-galactosidase activity measured in lysates of SR7 cultures that contain an empty pXyl plasmid or pXyllacZ. Activity was normalized to total protein concentration in the lysate to control for growth differences and differential cell lysis. Errors represent standard deviation of biological replicate cultures (n> 4). For cultures grown under 0.1 MPa CO2, overnight anaerobic cultures grown from spores were subcultured into CO2-evacuated vials to a uniform optical density. Induction with xylose occurred 2 h after subculture, and the time point for LacZ activity measurement was taken 4 h post induction. For cultures grown under 10 MPa scCO2, SR7 pXyllacZspores were loaded into stainless steel culture vessels with and without xylose inducer. Cultures were grown for 21 days and microscopy was used to determine which samples showed at least a tenfold increase in cell number prior to measuring LacZ activity. Source data are provided as aSource Datafile SR7 pXyl lacZ cultures amended with xylose grew in 8 of 55 columns (15%) while growth was observed in 5 of 34 unamended columns (15%) (Supplementary Table 3 ), which together represent a 4.4-fold decrease in growth frequency relative to wild-type SR7 (64%) under the same conditions (i.e., 5 ml culture volume with 3 × 10 5 spores ml –1 inoculum and 5 ml scCO 2 headspace) [25] . Previous studies have shown bacteria transformed with exogenous plasmids are more susceptible to cell death than wild-type strains, especially under harsh culture conditions [38] , [39] , consistent with our results. Improving growth of genetically modified SR7 remains an important target for further optimization. Alcohol production and optimization in aerobically grown SR7 An isobutanol bioproduction pathway was developed in SR7 due to previous success at achieving high yields and titers of this compound in B. subtilis [31] , [40] , and the fact that the isomer n -butanol can be effectively extracted from a biphasic aqueous-scCO 2 reactor [12] . Furthermore, isobutanol generation from 2-ketoisovelerate (αKIV) is expected to require heterologous expression of only one enzyme, α-ketoisovalerate decarboxylase (KivD from L. lactis ) [27] (Fig. 4a ), since the SR7 genome encodes eight predicted alcohol dehydrogenases [25] . For SR7 grown in LB medium under aerobic conditions, isobutanol production was only observed for cells that contained kivD , with approximately 50% yield on αKIV in cultures that were both induced with xylose and fed the αKIV substrate (Fig. 4b ). To increase product yield, the alcohol dehydrogenase ADH6 Sc from S. cerevisisae was overexpressed in tandem with KivD, resulting in approximately 70% yield of isobutanol on αKIV for xylose-induced cells (Fig. 4b ). In addition to the target isobutanol molecule, isopentanol (Fig. 4c and Supplementary Figs. 6 and 7 ) and phenylethyl alcohol (PEA) (Supplementary Fig. 8a ) production were also observed, with the isopentanol titer being greater than that of isobutanol. Accumulation of these products is not surprising given the known promiscuity of KivD towards other amino acid synthesis pathway intermediates [27] (Supplementary Fig. 8b ). Fig. 4 Isobutanol and isopentanol production in SR7. a Two-step enzyme pathway to convert the valine intermediate 2-ketoisovalerate (αKIV) to isobutanol using the decarboxylase enzyme KivD from L. lactis and an alcohol dehydrogenase. b Evaluation of isobutanol production at 24 h post induction in SR7 with an empty pXyl plasmid, pXyl kivD , pXyl kivD ADH6 Sc , or pXyl kivD yqhD Ec , where ADH6 and YqhD are alcohol dehydrogenases from S. cerevisiae and E. coli , respectively. Cultures were grown aerobically in LB medium in the presence and absence of 5 g l –1 xylose as an inducer and 5 mM αKIV as substrate for the pathway. For all aerobic experiments, error bars represent the standard deviation of biological triplicate cultures. c Co-production of isopentanol measured in SR7 samples shown in b . d Accumulation of the isobutyraldehyde intermediate at short culture times, 4 h post induction. Alcohol dehydrogenases ADH6 from S. cerevisiae , AdhA from L. lactis , AdhP from E. coli , YqhD from E. coli , and AdhA from B. megaterium SR7 were evaluated to decrease the buildup of isobutyraldehyde intermediate for aerobic cultures fed 5 mM αKIV and induced with xylose. e Production of isobutanol at 24 h post induction for the cultures shown in d . f Production of isobutanol for SR7 cultures grown under 0.1 MPa CO 2 (biological triplicate cultures) and 10 MPa scCO 2 at 37 °C. Under scCO 2 , cultures with at least a tenfold increase in cell number, as enumerated by microscopy, were analyzed for alcohol production, sugar consumption and fermentation product generation. Average isobutanol titers from the aqueous phase of cultures showing at least 1 mM glucose consumption (classified as high activity; Supplementary Fig. 11 ) are provided. Source data are provided as a Source Data file Full size image Biosynthesis of alcohols entails conversion of aldehyde intermediates (Fig. 4a ) that tend to be highly soluble in scCO 2 , partitioning approximately tenfold more readily into scCO 2 than their cognate alcohols [7] . Thus, any accumulation of aldehyde is hypothesized to result in premature extraction of this compound under scCO 2 , resulting in lower alcohol production. Under aerobic conditions at short induction times of 4 h, isobutyraldehyde buildup was observed, even for cells that contained the alcohol dehydrogenase ADH6 Sc (Fig. 4d ). Four additional alcohol dehydrogenases were screened for reduced aldehyde accumulation: three previously shown to be functional within the context of the isobutanol pathway [41] , and a predicted alcohol dehydrogenase native to SR7 (AdhA Bm ) with high homology to AdhA Ll from L. lactis . The YqhD enzyme from E. coli , known to be highly effective for producing isobutanol [41] , [42] , was identified as the superior variant, with the lowest amount of aldehyde accumulation at short culture times (4 h) (Fig. 4d ), over 80% yield of isobutanol from αKIV (Fig. 4e ), and maintained capacity for isopentanol production ( Fig. 4c ). The optimized two-enzyme isobutanol production pathway was evaluated aerobically in semi-defined medium containing 4 g l –1 glucose and 5 g l –1 xylose (conditions previously shown to support heterologous enzyme production in SR7 under anaerobic conditions). The final isobutanol titer was approximately half of that observed in LB medium (Supplementary Fig. 9a ), possibly due to lower heterologous enzyme expression and more αKIV substrate being directed towards biomass in the lower nutrient semi-defined medium. Increasing the glucose concentration to 10 g l –1 in the semi-defined medium increased the titers of all three alcohols, suggesting that cellular resources may be directed towards these products when carbon is provided in greater excess (Supplementary Fig. 9b ). When neither glucose nor xylose were supplied, minimal biomass (OD 600 < 0.1) or product accumulated (Supplementary Fig. 9c ), indicating that neither growth nor alcohol production is due to trace amounts of yeast extract (50 mg l –1 ). Xylose alone enabled high cell density growth (OD 600 > 6.5), and in the case of isopentanol, almost 1 mM production, with a further increase in titer upon adding αKIV substrate (Supplementary Fig. 9c ). When combined with xylose, the addition of 100 mM alanine (used under anaerobic CO 2 conditions for endospore germination) increased cell growth (OD 600 > 15) and more than doubled isobutanol production (Supplementary Fig. 9d ), likely due to the deamination of alanine to pyruvate, a precursor for isobutanol via the valine-synthesis pathway and part of central carbon metabolism. Isobutanol production in SR7 under scCO 2 After optimizing aldehyde conversion and alcohol production for SR7 under aerobic conditions, functionality of the two-step isobutanol pathway was assessed in semi-defined medium under anaerobic conditions (Fig. 4f ). Seed cultures of SR7 pXyl kivD yqhD Ec cells passaged under 0.1 MPa CO 2 into fresh medium amended with xylose and 5 mM αKIV substrate generated 4.43 mM isobutanol after 48 h of incubation. The final isobutanol titer under anaerobic 0.1 MPa CO 2 headspace is greater than the 2 mM isobutanol generated by aerobic cells grown in the same medium conditions. Isopentanol and PEA titers were 1.8 and 0.21 mM, respectively (Supplementary Fig. 10 ). As expected, no isobutanol or isopentanol was observed for SR7 cultures that contained an empty plasmid (Fig. 4f and Supplementary Fig. 10 ). Biofuel production was next evaluated for SR7 cultures grown under supercritical CO 2 at 10 MPa and 37 °C. Cultures were grown for 21 days in semi-defined medium from SR7 endospores containing the desired biofuel pathway or empty plasmid, with 4 g l –1 glucose, 5 g l –1 xylose, 5 mM αKIV, and 100 mM alanine added at the time of inoculation. As was found for SR7 pXyl lacZ , the addition of a plasmid resulted in lower frequency growth (27%) as compared to SR7 wild-type (64%) [25] (Supplementary Table 3 ). For cultures that displayed growth, glucose consumption was not correlated with increases in cell number (Supplementary Fig. 11a ), possibly due to consumption of yeast extract and l -alanine. Glucose consumption was found to correlate strongly with the production of fermentation products lactate and acetate ( R 2 = 0.97) (Supplementary Fig 11b ), which have previously been shown to accumulate in SR7 cultures grown under scCO 2 [25] . This finding led to classifying samples that consumed more than 1 mM glucose as having high activity, as all of these samples also produced greater than 1 mM combined lactate and acetate (Supplementary Fig. 11b ). Other samples that showed at least tenfold growth, but less than 1 mM glucose consumption were classified as having low activity since they neither consumed sugar substrate nor generated meaningful amounts of fermentation products (Supplementary Fig. 11b ). Isobutanol production was measured from the aqueous phase of scCO 2 cultures grown in the presence and absence of xylose (Supplementary Fig. 12 ). Xylose-containing high activity cultures produced an average of 1.23 mM isobutanol, whereas those without xylose generated approximately half that amount (Fig. 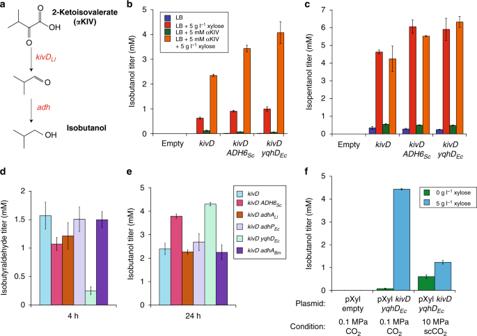Fig. 4 Isobutanol and isopentanol production in SR7.aTwo-step enzyme pathway to convert the valine intermediate 2-ketoisovalerate (αKIV) to isobutanol using the decarboxylase enzyme KivD fromL. lactisand an alcohol dehydrogenase.bEvaluation of isobutanol production at 24 h post induction in SR7 with an empty pXyl plasmid, pXylkivD, pXylkivD ADH6Sc, or pXylkivD yqhDEc, where ADH6 and YqhD are alcohol dehydrogenases fromS. cerevisiaeandE. coli, respectively. Cultures were grown aerobically in LB medium in the presence and absence of 5 g l–1xylose as an inducer and 5 mM αKIV as substrate for the pathway. For all aerobic experiments, error bars represent the standard deviation of biological triplicate cultures.cCo-production of isopentanol measured in SR7 samples shown inb.dAccumulation of the isobutyraldehyde intermediate at short culture times, 4 h post induction. Alcohol dehydrogenases ADH6 fromS. cerevisiae, AdhA fromL. lactis, AdhP fromE. coli, YqhD fromE. coli, and AdhA fromB. megateriumSR7 were evaluated to decrease the buildup of isobutyraldehyde intermediate for aerobic cultures fed 5 mM αKIV and induced with xylose.eProduction of isobutanol at 24 h post induction for the cultures shown ind.fProduction of isobutanol for SR7 cultures grown under 0.1 MPa CO2(biological triplicate cultures) and 10 MPa scCO2at 37 °C. Under scCO2, cultures with at least a tenfold increase in cell number, as enumerated by microscopy, were analyzed for alcohol production, sugar consumption and fermentation product generation. Average isobutanol titers from the aqueous phase of cultures showing at least 1 mM glucose consumption (classified as high activity; Supplementary Fig.11) are provided. Source data are provided as aSource Datafile 4f and Supplementary Table 4 ). 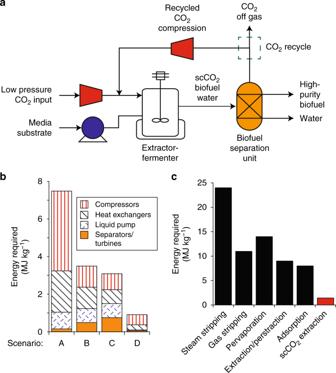Fig. 5 Isobutanol energy recovery requirements for integrated fermentation-extraction under scCO2.aSimplified process schematic of the envisioned scCO2bioprocess used to develop an Aspen Plus model, including compression of CO2to scCO2, fermentation/extraction, de-pressurization/biofuel recovery, and CO2recycle. Further detail is provided in Supplementary Fig.15a.bEnergy requirement for isobutanol recovery as MJ kg−1for several scenarios. Separate fermentation and scCO2recovery processes represent the base case (scenario A). Scenario B is coupled fermentation and extraction without use of partial extraction stream de-pressurization or scCO2recycle. Scenario C de-pressurizes the extraction stream to 6.5 MPa to induce formation of an isobutanol-rich stream, which permits recycling of compressed CO2, set at 50% (by mass). Scenario D again de-pressurizes to 6.5 MPa and recycles the maximum possible amount of CO2(87%) that results in no accumulation of CO2in the system. Values forbcan be found in Supplementary Table6.cComparison of the energy requirements for isobutanol production found for the scCO2process relative to published literature values for alternative in situ recovery methods28. The scCO2extraction energy requirement incis for coupled fermentation and extraction with partial de-pressurization and full recycle (i.e., Scenario D inb). Source data are provided as aSource Datafile Isobutanol titers normalized to cell density were comparable under 0.1 MPa CO 2 and 10 MPa scCO 2 , at 2.2 × 10 –8 μmol cell –1 and 3.1 × 10 –8 μmol cell –1 , respectively (Supplementary Table 5 ). While the high activity, empty vector control cultures consumed up to 1.9 mM αKIV under 10 MPa scCO 2 , isobutanol was not detected in any of these samples (Supplementary Table 4 ), an identical outcome to aerobic and 0.1 MPa CO 2 cultures. The isobutanol yield from αKIV ranged from 37 to 45% in the aqueous phase for xylose-induced high activity biofuel cultures, 2.8-fold higher than for those that lacked xylose (Supplementary Table 4 ). Isopentanol generation was also observed for samples grown under 10 MPa scCO 2 , reaching an average titer of 0.31 mM (Supplementary Table 4 ), while only trace amounts of PEA were detected under scCO 2 . The amount of isobutanol produced by low activity cultures was on average 35-fold less than for the high activity cultures (Supplementary Table 4 ). Extraction of isobutanol using scCO 2 Inspired by our demonstration of microbially generated alcohols under scCO 2 , we attempted to recover product from SR7 cultures using scCO 2 . Partitioning of biologically produced isobutanol into the scCO 2 headspace was observed for the aforementioned SR7 cultures (Supplementary Fig. 13 ), albeit at marginal concentrations. Isopentanol was not detected in the headspace samples. Our proof of concept demonstration for isobutanol extraction motivates adoption of two engineering solutions to increase recovery: (1) use of flowing scCO 2 to increase mass transfer and (2) controlled de-pressurization to capture scCO 2 -solubilized alcohol. To evaluate these solutions, we assessed the recovery of isobutanol in the absence of microbial cells using a stirred two-phase reactor that is designed for in situ extraction using scCO 2 stripping (Supplementary Fig. 14 ), as previously done for n- butanol and n -pentanol [12] . Similar to straight-chained alcohols, the rate of isobutanol extraction from aqueous solutions increases with low scCO 2 flow rates, reaching a maximum at a flow rate of 3.2 ml min –1 , most likely due to a tradeoff between convective and diffusive mass transfer. Isobutanol extraction rate and efficiency using scCO 2 was found to be approximately 25% greater than that for n -butanol (Supplementary Fig. 14 ). Taken together, these data indicate that scCO 2 is effective for rapid extraction of isobutanol from dilute aqueous solutions and identifies scale up of cultures to a similarly designed system as a priority for further development. Process analysis for extraction using scCO 2 The experimental component of this study established growth and heterologous bioproduction in the presence of scCO 2 and extraction of isobutanol into the scCO 2 phase in a stirred reactor. Next, we constructed a fermentation-extraction process model to assess technological potential using detailed mass and energy balances. The objective of the analysis was calculation of isobutanol recovery energy requirements for comparison with previously reported analyses of butanol recovery using other methods [28] . In practice, Oudshoorn suggested a benchmark of 5 MJ kg –1 as the maximum energy requirement for butanol recovery [28] . Unfortunately, previous studies of butanol recovery from dilute fermentation broths ( < 20 g l –1 ) using a wide range of conventional technologies, such as gas stripping, adsorption, and liquid–liquid extraction, report energy requirements in the range of 10–20 MJ kg –1 [28] . By comparison, Tompsett et al. [12] estimated the energy demand for the CO 2 compression required for scCO 2 extraction of dilute n -butanol to be 4.0 MJ kg –1 . Since CO 2 compression is expected to represent the majority of the energy required by the scCO 2 extraction process, these results [12] suggest that the energy requirement of scCO 2 extraction might compare favorably with alternative technologies — especially since efforts to minimize CO 2 compression requirements were not considered. Moreover, this previous study [12] did not analyze the performance of an integrated fermentation-extraction process since bioproduction in the presence of scCO 2 has never been reported prior to this work. Accordingly, the current study evaluated approaches to reduce CO 2 compression requirements, the advantages associated with coupled fermentation-extraction (Supplementary Note 3 ), and the intrinsic performance of the scCO 2 extraction process. With emphasis on evaluating energy demand for recovering a high-purity product, we developed an Aspen Plus simulation model (Fig. 5a and Supplementary Fig. 15a ) to analyze a process consisting of integrated fermentation and extraction using scCO 2 . Isobutanol extraction performance was simulated using data reported in the current work, literature data on n -butanol extraction [12] , [43] , [44] , and established thermodynamic properties [45] , [46] (Supplementary Note 3 ). Sensitivity analysis revealed that the most influential parameter in determining isobutanol energy requirement was the CO 2 :isobutanol feed ratio since it directly relates to the amount of CO 2 that must be compressed for extraction (Supplementary Fig. 15b and Supplementary Note 3 ). Combining our isobutanol extraction data with values reported on n- butanol [44] , we calculate that 99.73% isobutanol recovery could be achieved at a CO 2 :isobutanol feed ratio of 3:1 as a base case. To reduce CO 2 compression energy demand, product recovery via partial de-pressurization of the CO 2 stream was explored, finding > 94% pure isobutanol product could be recovered by partially de-pressurizing the stream exiting the fermenter to between 3.5 and 6.5 MPa [45] . In this pressure range, liquid–liquid phase splitting occurs, resulting in isobutanol-rich and water-rich liquids [45] . Partial de-pressurization allows recycling of a high-pressure CO 2 stream, further reducing CO 2 compression demand and thereby energy consumption (Supplementary Fig. 15b ). Lastly, the sensitivity of the process to the ratio of recycled to purged CO 2 was investigated using an optimized intermediate pressure of 6.5 MPa (Supplementary Fig. 15b ). Increasing the CO 2 recycle amount decreased energy requirements nearly linearly, with the best performance observed at the limit of 87% recycle (Supplementary Fig. 15c ). Fig. 5 Isobutanol energy recovery requirements for integrated fermentation-extraction under scCO 2 . a Simplified process schematic of the envisioned scCO 2 bioprocess used to develop an Aspen Plus model, including compression of CO 2 to scCO 2 , fermentation/extraction, de-pressurization/biofuel recovery, and CO 2 recycle. Further detail is provided in Supplementary Fig. 15a . b Energy requirement for isobutanol recovery as MJ kg −1 for several scenarios. Separate fermentation and scCO 2 recovery processes represent the base case (scenario A). Scenario B is coupled fermentation and extraction without use of partial extraction stream de-pressurization or scCO 2 recycle. Scenario C de-pressurizes the extraction stream to 6.5 MPa to induce formation of an isobutanol-rich stream, which permits recycling of compressed CO 2 , set at 50% (by mass). Scenario D again de-pressurizes to 6.5 MPa and recycles the maximum possible amount of CO 2 (87%) that results in no accumulation of CO 2 in the system. Values for b can be found in Supplementary Table 6 . c Comparison of the energy requirements for isobutanol production found for the scCO 2 process relative to published literature values for alternative in situ recovery methods [28] . The scCO 2 extraction energy requirement in c is for coupled fermentation and extraction with partial de-pressurization and full recycle (i.e., Scenario D in b ). Source data are provided as a Source Data file Full size image Based on these sensitivity analyses, four scenarios were assessed using the process model, with specific emphasis on evaluating the extent to which partial de-pressurization and CO 2 recycling could be used to decrease energy requirements of isobutanol extraction (Fig. 5b and Supplementary Table 6 ). Atmospheric-pressure fermentation followed by scCO 2 extraction (scenario A) required an estimated 6.80 MJ kg –1 , with compression accounting for approximately 66% of the energy demand. An integrated process, with complete de-pressurization to 0.1 MPa and no CO 2 recycling (scenario B), reduced the energy burden to 4.4 MJ kg –1 , with most of the improvement stemming from reduced compression requirements. Intermediate de-pressurization to 6.5 MPa combined with 50% CO 2 recycle (scenario C) [43] , further reduces the energy requirement to 2.4 MJ kg –1 , again largely due to diminished compression requirements. Finally, placing the CO 2 recycle ratio at its maximum value (87%) (scenario D) and de-pressurizing the extraction stream to 6.5 MPa reduces the energy requirement to 1.4 MJ kg –1 . As expected from previous arguments, the newly established energy requirement is lower than that previously reported for stand-alone fermentation and scCO 2 extraction, and much less than any figure reported for conventional technologies such as gas stripping, liquid–liquid extraction, or adsorption (Fig. 5c ). Although the energy requirement estimated here for integrated extraction-fermentation has not yet been demonstrated in practice, the current finding motivates further evaluation, with our model serving as a basis for follow-on techno-economic, emissions, and life cycle assessment studies. In this work, we report the production of alcohol biofuels under supercritical carbon dioxide. Using an environmentally isolated strain ( Bacillus megaterium SR7) native to a deep subsurface CO 2 reservoir, a transformation protocol was developed and heterologous protein expressed from three promoters. Furthermore, inducible β-galactosidase production was observed for cells grown under scCO 2 . SR7 was engineered to produce isobutanol from αKIV through a two-step metabolic pathway that simultaneously produced isopentanol. Both isobutanol and isopentanol have potential as drop-in biofuels or fuel additives, with comparable energy densities (29 MJ l –1 and 28 MJ l –1 , respectively) and research octane numbers (98 and 105) [47] . Similar to isobutanol, isopentanol is predicted to be highly miscible in scCO 2 [12] . For cultures grown under scCO 2 that showed high activity, isobutanol titers were greater than 1 mM, with 42% average yield on consumed αKIV substrate. Importantly, while total titers were reduced at 10 MPa, specific titers under scCO 2 were similar to those observed under 0.1 MPa conditions, at 2.2 × 10 −8 μmol cell –1 and 3.1 × 10 −8 μmol cell –1 , respectively. Recovery of microbially generated isobutanol using scCO 2 was demonstrated, but limited, due to both the configuration of the high-pressure culturing vessels and the low titers achieved. Separation of dilute isobutanol from aqueous media using scCO 2 is possible using a two-phase extractor-fermenter, as previously observed for straight-chain alcohols [12] . Lastly, process analysis shows that using scCO 2 to extract biofuels is energetically feasible and comparable, if not better, than other in situ extraction techniques if sufficiently high product titers can be achieved. As such, this work serves as a starting point for bioproduction under scCO 2 with numerous avenues for continued optimization. Further development of the genetic toolbox for SR7 will enable future metabolic engineering of SR7 for enhanced biochemical production. Isobutanol pathway optimization was briefly explored by screening five alcohol dehydrogenases and selecting the variant that resulted in highest substrate conversion ( > 80%) and minimal aldehyde accumulation at short incubation times. Additionally, isopentanol and phenylethyl alcohol production were observed through the simple addition of a decarboxylase, possibly due to upregulation of the leucine and phenylalanine synthesis pathways in SR7. Other strains of B. megaterium are known to accumulate the amino acids lysine [48] and possibly valine [49] ; however, evidence for leucine and phenylalanine accumulation was not previously observed [49] . The leucine biosynthesis pathway may become a starting point for future engineering efforts to increase isopentanol titers or make additional bioproducts due to the already presumably high flux of the pathway [50] . To ensure that coupled fermentation-extraction technology is utilized to its full potential, initial screening of subsequent compounds to be made by SR7 will be determined based on their preferential partitioning into scCO 2 and toxicity to bioproduction hosts. Taking advantage of scCO 2 for properties beyond its well-established extractive [12] and sterilizing capabilities [13] would confer additional utility to this technology. For example, scCO 2 has been used for the depolymerization of lignocellulosic biomass to release fermentable sugars [51] . Combining the two technologies could provide an inexpensive substrate for SR7 growth and bioproduction. Carboxylation reactions may also be possible in SR7, directly using CO 2 or HCO 3 – found in solution for bioproduction [52] , [53] . Even with the low solubility of scCO 2 in water [54] , the approximate HCO 3 – concentration of 1.1–1.3 mM (based on Henry’s law and the reaction of CO 2(aq) with water) is advantageous relative to other studies that use air as a CO 2 source for carbon fixation through heterologous overexpression of a carboxylase [55] , [56] . SR7 contains several predicted carboxylases, including pyruvate carboxylase, two PEP carboxylases and a biotin-dependent acetyl-CoA carboxylase, each of which could serve as pathways to route HCO 3 – into central carbon metabolism [25] . Additionally, the SR7 genome encodes two predicted carbonic anhydrases for converting CO 2(aq) to HCO 3 – . Lastly, Bacillus megaterium strains are known for their ability to secrete proteins [57] , conferring further biotechnological utility to this host for ex vivo reactions. One of the limitations to using scCO 2 for bioprocessing is the slow and infrequent growth observed for SR7, especially when bearing an exogenous plasmid. Significant improvements were previously made for scCO 2 culturing using SR7 through media optimization and recognition of endospore germination as a key step for acclimation of this strain to conditions associated with scCO 2 exposure [25] . Future work will be conducted to better understand the factors limiting growth of SR7 under scCO 2 and to select for strains of SR7 that demonstrate more robust and rapid outgrowth into vegetative cells. Enhanced understanding and substantial improvement of SR7 growth will similarly inform economic, environmental, and energy analysis of the integrated process, due to the inter-relationships between growth, productivity, titer, scCO 2 volumes and extraction efficiency, energy requirements, and ultimately cost. Numerous studies have shown the ability to improve the tolerance of microbes to harsh environments, including through the use of adaptive laboratory evolution [58] . Many of these studies, however, found that increased tolerance of strains does not necessarily correlate with enhanced specific titers when used for bioproduction [59] , [60] , [61] . For SR7, the fact that specific titer is comparable under atmospheric and scCO 2 conditions suggests that scCO 2 does not impair specific productivity and that improvements in titer observed under 1 atm CO 2 will positively translate into higher titers under scCO 2 . Using the plasmid bearing strains in this work, future selection of SR7 mutants that have a higher growth capacity despite the burden associated with plasmid maintenance and expression may also be possible [62] . Additionally, genomic integration could alleviate plasmid-maintenance burden for SR7 strains, and recently developed Cas9-based genomic modification strategies for B. subtilis strains [63] , [64] provide a starting point for integrating and removing desired and competing pathways, respectively, in SR7. The isolation, characterization and genetic engineering of an scCO 2 -tolerant strain of B. megaterium establishes exciting biotechnological opportunities for in vivo high-pressure CO 2 bioprocessing coupled with in situ product extraction. While low-frequency growth from Bacillus spp. spores [22] and enzymatic catalysis [15] have previously been shown under scCO 2 , this work demonstrates combined heterologous enzyme expression and bioproduct synthesis under these harsh conditions. Proven scCO 2 stripping of biofuels and favorable energy requirements of scCO 2 -based bioprocessing lend credibility to the adoption of this process for commercial applications, motivating continued work to improve titers, yields, and productivities. Achieving such improvements would enable demonstration of the integrated extraction-fermentation process at a larger scale, facilitating collection of data needed to form the basis for full techno-economic and life cycle analyses, and more detailed comparisons to other extraction strategies and renewable energy sources. Plasmid construction For plasmid construction (Supplementary Table 7 ), restriction enzymes, T4 DNA ligase, and Q5 High-Fidelity PCR MasterMix were purchased from NEB and used according to manufacturer recommendations. The pXyl gfp plasmid is based on the pRBBm34 shuttle vector [65] (purchased from Addgene), which contains a xylose-inducible promoter, the xylose repressor ( xylR ) under control of its native B. megaterium promoter, ampicillin resistance marker (Amp r ) for selection in E. coli , tetracycline resistance marker (Tet r ) for selection in B. megaterium , and two origins of replication. The gene encoding SuperFolder GFP was PCR amplified from the pTRC99a gfp SF (lab stock) template using the oligonucleotides Spe I gfp for and gfp Sph I rev (Supplementary Table 8 ). The resulting PCR product and pRBBm34 plasmid were digested with Spe I and Sph I, and resulting fragments ligated to create pXyl gfp . The pXyl empty plasmid was generated by adding the DNA sequence 5ʹ-atttaatgttgatgaaagctggtctggtgtcaaaaataatga-3ʹ between the Spe I and Sph I restriction enzyme sites. Ligated plasmid products were used to transform DH5α and plated on LB agar containing 100 μg ml –1 carbenicillin (Sigma). Plasmids were purified (Zippy plasmid miniprep kit, Zymo research) prior to verification by DNA sequencing (Genewiz) using appropriate sequencing oligonucleotide primers (Supplementary Table 8 ). The xylose repressor and promoter of pRBBm34 were replaced with a hyperspank promoter and lacI using circular polymerase extension cloning (CPEC). The pRBBm34 plasmid was PCR linearized with two sets of primers to remove xylR and the xylose promoter: pRBBm34 for/ bla rev and bla for/pRBBm34 rev. The hyperspank promoter and lacI were PCR amplified from pDR111 [66] (gift from Alan Grossman, MIT Department of Biology) using primers pRBBm34-pHysp for and lacI -pRBBm34. A standard CPEC protocol [67] was used to assemble the three PCR products into the pHysp empty plasmid. Gfp was PCR amplified from pXyl gfp using primers Sal I RBS gfp for and gfp Nhe I rev. The gfp PCR product and pHysp empty were digested with Sal I and Nhe I, and the fragments were assembled to make pHysp gfp . To generate the p43 empty and p43 gfp plasmids, the pXyl empty and pXyl gfp plasmid (respectively) were PCR linearized with oligonucleotide sets RBS-start for/ bla rev and bla for/pRBBm34 rev. The p43 promoter was PCR amplified from Bacillus subtilis strain KS438 using primers pRBBm34-p43 for and p43-RBS-start rev. The two p43 plasmids were created by assembling the three PCR fragments using CPEC. All the remaining plasmids were made using standard restriction enzyme digest and ligation construction; the pairs of restriction enzymes used are indicated in the oligonucleotide primer names. The gene encoding β-galactosidase from E. coli was PCR amplified from the plasmid pKVS45 lacZ _LVA (lab stock) using primers Spe I lacZ Ec for and lacZ Ec Sph I rev. The ketoisovalerate decarboxylase gene from L. lactis was amplified from pCOLA (Fjoh-2967) ( kivD ) [68] with primers Spe I kivD Ll for and kivD Ll Bam HI Sph I rev for the construction of pXyl kivD Ll . The ADH6 gene from Saccromyces cerevisiae was amplified from pACYC ( car sfp ) ( ADH6 Sc ) [68] using primers Bam HI RBS ADH6 Sc for and ADH6 Sc Sph I rev to make the plasmid pXyl kivD Ll ADH6 Sc . For all the alcohol dehydrogenases studied, the RBS 5ʹ-agggggaaa-3ʹ was used. The adhA Ll gene was amplified from the L. lactis subsp. lactis (ATCC 19435D) genome (primers: Bam HI adhA Ll for and adhA Ll Sph I rev), adhP Ec and YqhD Ec from the E. coli MG1655 genome (primers: Bam HI adhP Ec for and adhP Ec Sph I rev; Bam HI yqhD Ec for and yqhD Ec Sph I rev, respectively), and adhA Bm from the B. megaterium SR7 geneome (primers: Bam HI adhA Bm for and adhA Bm Sph I rev). All alcohol dehydrogenases were ligated between the Bam HI and Sph I sites in pXyl kivD Ll . Transformation of SR7 and verification Protoplast transformation of SR7 was adapted from an established method by Biedendieck et al. [29] . All buffers described in this protocol were identical to those in Biedendieck et al. [29] and were made with chemicals from Millipore-Sigma unless otherwise described. An overnight culture of SR7 was grown from the inoculation of 50 ml of LB medium (BD Difico) with a single SR7 colony, and was incubated at 37 °C and 250 r.p.m. SR7 was subcultured at a dilution of 1:100 in fresh LB medium and grown at 37 °C and 250 r.p.m. until an OD 600 reading of 1.0 was reached (~3 h) (Implen NanoPhotometer). Cells were collected by centrifugation at 4000 × g for 10 min and the cell pellet was retained. The cell pellet was resuspended in 5 ml 1x SMMP buffer (2.32 g l -1 L -malic acid (Alfa Aesar), 1.6 g l -1 NaOH, 4.06 g l -1 MgCl 2 •6H 2 0, 171.16 g l -1 sucrose, 17.5 g l -1 antibiotic medium number 3 (AB3) (BD Difico)). Lysozyme (Sigma) was added to a concentration of 30 μg ml –1 , which was tenfold lower than used in previous methods [29] . Protoplast formation was performed at 37 °C for 10 min at 70 r.p.m. and was visualized by microscopy. Protoplasts were collected by centrifugation at 1300 r.p.m. for 10 min, followed by a wash with 5 ml 1x SMMP. Protoplasts were resuspended gently in 5 ml 1x SMMP and were aliquoted into 0.5 ml fractions. Each sample was transformed with 3 μg freshly prepared plasmid DNA (Zippy plasmid miniprep kit, Zymo research) and 1.5 ml of a 20% PEG 8000 (Promega) solution in 1x SMM (2.32 g l -1 L -malic acid (Alfa Aesar), 1.6 g l -1 NaOH, 4.06 g l -1 MgCl 2 •6H 2 0, 171.16 g l -1 sucrose). Samples were incubated with gentle mixing for 2 min, followed by addition of 5 ml 1x SMMP and centrifugation to collect the transformed protoplasts. The protoplasts were resuspended in 0.5 ml 1x SMMP and incubated at 37 °C for 1.5 h at 100 r.p.m. to recover. Transformed protoplasts were plated in a soft agar overlay [29] on dried and pre-warmed LB agar plates containing 5 μg ml –1 tetracycline (Calibiochem). Additionally, protoplasts were plated in agar overlays on LB agar without antibiotic to determine viability. Plates were incubated for two days at 30 °C. Confirmation of SR7 transformation was carried out using several techniques including colony PCR, streaking colonies on fresh LB agar plates containing 5 μg ml –1 tetracycline, sequencing isolated plasmid DNA, and back transforming plasmid DNA into E. coli . For colony PCR, colonies were picked and boiled for 10 min to serve as template for the PCR reaction using OneTaq Quick-Load Master Mix (NEB) and appropriate sequencing primers (Supplementary Table 8 ). Plasmid DNA was isolated from SR7 using a standard plasmid isolation protocol and materials (Zippy plasmid miniprep kit, Zymo research), except 10 μg ml –1 lysozyme was added for the initial resuspension step with a 1 h incubation at 37 °C to promote cell lysis. Standard Sanger sequencing of isolated plasmids was used to verify identity (Genewiz). Purified plasmids were also backtransformed into E. coli DH5α, which were subsequently plated on LB agar containing 100 μg ml –1 carbenicillin. Plasmid stability was assessed by isolating the backtransformed plasmid DNA and restriction enzyme digestion with Eco RI (NEB). For a positive control, purified pXyl gfp directly from E. coli DH5α was also digested with Eco RI. Lastly, SR7 species and strain identity was confirmed through preparation of genomic DNA (Wizard genomic DNA purification kit, Promega) and sequencing of the PCR amplified 16s rRNA and xylE genes, respectively. The 16s fragment was PCR amplified using Q5 High-Fidelity MasterMix (NEB) and the 27F and 1492R primers (Supplementary Table 8 ); the xylE gene was amplified using xylE Bm seq for and xylE Bm seq rev primers. Aerobic SR7 culturing SR7 was cultured aerobically in complex LB medium and a semi-defined M9-based medium. The semi-defined medium consisted of 1x M9 salts (Sigma) (7 g l –1 Na 2 HPO 4 •7H 2 O, 3 g l –1 KH 2 PO 4 , 0.5 g l –1 NaCl, 1 g l –1 NH 4 Cl), 2 mM MgSO 4 , 0.04 mM MgCl 2 , 0.05 g l –1 yeast extract (BD Difico), 1x trace metals supplement [69] (5 mg l –1 Na 2 (EDTA), 0.2 mg l –1 NiSO 4 •6H 2 O, 0.5 mg l –1 CoCl 2 •6H 2 O, 0.1 mg l –1 H 2 FeO 3 , 1 mg l –1 FeSO 4 •7H 2 O, 0.1 mg l –1 H 3 BO 3 , 1 mg l –1 ZnCl 2 , 0.1 mg l –1 NaMoO 4 •2H 2 O, 0.4 mg l –1 AlCl 3 •6H 2 O, 1 mg l –1 MnCl 2 •4H 2 O, 0.3 mg l –1 Na 2 NO 4 •2H 2 O, 0.2 mg l –1 CaCl 2 ), and desired concentration of glucose or xylose. For SR7 strains that contained a plasmid, the medium was amended with 5 μg ml –1 tetracycline. Overnight cultures were started in desired medium by picking colonies from freshly grown LB agar plates with 5 μg ml –1 tetracycline; different colonies were selected for experiments performed in biological triplicate. Overnight cultures (5 ml) were incubated for approximately 16 h at 37 °C and 250 r.p.m.. For gfp production, SR7 was subcultured into 1 ml of fresh medium using 20 μl of an overnight culture into a 48-well flower-plate (m2p labs). Plates were sealed with porous adhesive film for culture plates (VWR) to reduce evaporation, and cultures were grown in a BioLector (m2p labs) at 1200 r.p.m., 37 °C, and 80% humidity. The BioLector continuously monitored (15 min cycle) OD and GFP fluorescence. OD measurements from the BioLector were converted to OD 600 measurements with a standard pathlength of 1 cm by generating a standard curve using exponentially grown SR7 cells and comparing a dilution series on the BioLector and Implen spectrophotometer. Protein induction occurred 3 h after subculturing (OD 600 ~0.4) by adding xylose to a final concentration of 5 g l –1 for strains that contain the pXyl plasmid, and IPTG to 1 mM for strains containing the pHysp plasmid. For alcohol production experiments, identical medium and starter culture procedures were used. Overnight cultures were subcultured to an OD 600 of 0.05 into 3 ml fresh medium in a 50 ml screw-capped tube (Pyrex) to avoid loss of volatile compounds. Protein induction occurred when the OD 600 of the culture reached approximately 0.4 by adding xylose to a final concentration of 5 g l –1 for strains that contain the pXyl plasmid. At the time of induction, αKIV was added to a final concentration of 5 mM. Alcohol production and isobutyraldehyde intermediate accumulation was measured 24 h and 4 h post induction, respectively. Cultures were centrifuged at 21,000 × g for 5 min to obtain cell-free supernatants. Alcohols and isobutyraldehyde were extracted from the cell-free supernatant using a 1:1 ratio of GC-grade ethyl acetate (Sigma), vortexing vigorously for 5 min, centrifuging at 21,000 × g for 5 min, and recovering the ethyl acetate fraction. Plasmid maintenance For plasmid maintenance studies, a 25 ml culture of SR7 pXyl gfp was grown in LB medium with 5 μg ml –1 tetracycline in a 250 ml baffled flask. Cultures were inoculated with 250 μl of an overnight culture and were subsequently incubated at 37 °C and 250 r.p.m. Protein induction occurred at 3 h post subculture using 5 g l –1 xylose. For each time point, an OD 600 reading was recorded, and cells were diluted to a uniform OD 600 in a black-lined 96-well plate (Costar) using LB medium prior to reading GFP fluorescence on a plate reader (Tecan infinite f200 pro, ex: 485/20 nm, em: 535/25 nm). To confirm plasmid maintenance at 74 h post induction, dilutions of cells were made in 1x M9 salts and were plated on LB agar with and without 5 μg ml –1 tetracycline to determine colony forming units. Colony PCR was performed using primers RepU seq for and RepU seq rev to amplify the RepU fragment, and primers pXyl seq for and gfp seq rev to amplify gfp (Supplementary Table 8 ). A negative control PCR reaction did not contain DNA template and a positive control used 1 ng μl –1 purified pXyl gfp . FACS and microscopy Samples for fluorescence activated cell sorting (FACS) were collected 4 h post induction for cells (or 7 h total culturing time for p43-containing cells) grown aerobically in LB medium as described above. Samples were prepared for FACS by diluting 5 μl of culture into 200 μl 1x M9 salts in a 96-well plate. FACS measurements were performed on a FACS Canto (BD) equipped with a high-throughput sampler, and GFP fluorescence was recorded from 488 nm emission laser coupled with the 530/30 nm filter channel. Populations of wild-type SR7 and SR7 with pXyl grown aerobically in LB medium were used to establish forward and side scatter gates to select events corresponding to the morphology of SR7. Fluorescence data was collected for 10,000 cell events for each sample. FACS data was analyzed using FlowJo software and a GFP positive gate was established for fluorescence values above all the negative control samples where SR7 contained an empty plasmid. Samples for microscopy of SR7 expressing gfp were also collected 4 h post induction for cultures grown aerobically in LB medium. Each sample was prepared as a wet-mount on a glass slide below a cover slip that had been prepared with poly- l -lysine (Sigma) to enable cells to adhere. Cells were visualized at 1000x magnification using an epifluorescence microscope (Zeiss Axioscope 2). Cell morphology was observed using phase-contrast microscopy and GFP fluorescence was visualized using a 480/30 nm excitation and 535/40 emission FITC filter set with a 505 nm long pass mirror and an X-Cite Series 200 fluorescence source. Images were captured on a Nikon D100 camera using the NKRemote live-imaging software. SR7 endospore preparation Overnight cultures of SR7 grown in LB medium aerobically were diluted 1:50 in modified G medium (2 g l –1 yeast extract, 2 g l –1 (NH 4 ) 2 SO 4 , 0.025 g l –1 CaCl 2 •2H 2 O, 0.5 g l –1 K 2 HPO 4 , 0.2 g l –1 MgSO 4 •7H 2 O, 0.05 g l –1 MnSO 4 •4H 2 O, 0.005 g l –1 ZnSO 4 •7H 2 O, 0.005 g l –1 CuSO 4 •5H 2 O, 0.0005 g l –1 FeSO 4 •7H 2 O, pH 7.1). For SR7 cells that contain a plasmid, both the vegetative cell growth medium and sporulation medium were supplemented with 5 μg ml –1 tetracycline. Sporulation was induced by incubating cutures in modified G medium for 72 h at 37 °C. Endospores were collected by centrifugation at 4000 × g and 4 °C for 15 min, and sporulation medium was removed by washing 5–10 times with cold wash buffer (0.058 g l –1 NaH 2 PO 4 •H 2 O, 0.155 g l –1 Na 2 HPO 4 •7H 2 O, 0.01% (vol/vol) Tween 20. Spore preparations were treated at 80 °C for 10 min to kill vegetative cells, and colony forming units were determined pre- and post-heat inactivation. Spore preparations were stored in wash buffer at 4 °C until use [22] . SR7 growth under 0.1 MPa CO 2 and 10 MPa scCO 2 Prior to anaerobic culturing, SR7 strains were prepared as endospores [22] . For cultures under 0.1 MPa CO 2 or 10 MPa scCO 2 , a semi-defined M9-based medium consisting of 1x M9 salts, 2 mM MgSO 4 , 0.04 mM MgCl 2 , 0.05 g l –1 yeast extract, 0.1x trace metals supplement, and 4 g l –1 glucose was degassed with CO 2 (Air gas) prior to use. Additionally, the medium was supplemented with 0.25 g l –1 of reducing agent Na 2 S and 1 mg l –1 of the redox indicator resazurin. All anaerobic culture manipulation occurred in an anaerobic chamber (Coy labs) under 0.1 MPa CO 2 . For low-pressure anaerobic experiments, SR7 cultures were grown under 0.1 MPa CO 2 headspace in 10 ml of CO 2 -degassed semi-defined medium in 100 ml serum vials with clamped rubber stoppers. Seed cultures were started by inoculating the degassed media in serum vials with 100 μl of previously prepared endospores; for SR7 samples that contain a plasmid, 0.5 μg ml –1 tetracycline was added. Cultures were grown for approximately 24 h at 37 °C and 250 r.p.m. Anaerobically grown vegetative cells were passaged into 10 ml of fresh medium to an OD 600 of 0.05. Cultures were incubated at 37 °C and 250 r.p.m., and protein expression was induced using a final concentration of 5 g l –1 xylose 2 h post subculture. For β-galactosidase production experiments, a 1 ml sample was taken 24 h after induction and centrifuged at 21,000 × g for 5 min, and cell pellets were retained and stored at –20 °C until analysis. For biofuel generation protocols, 5 mM αKIV was also added at the time of induction. Alcohols were collected 48 h post induction by centrifuging samples at 21,000 × g for 5 min and extracting the alcohols using ethyl acetate as was done for the aerobic samples. For 10 MPa scCO 2 cultures, M9 semi-defined medium was amended with 100 mM l -alanine (Sigma) to promote germination under pressure [25] . Samples were inoculated with endospores to a final concentration of 3 × 10 5 spores ml –1 . Xylose was added to a final concentration of 5 g l –1 for cultures to be induced, and αKIV to 5 mM for those to produce biofuels. As described in previous work [22] , high-pressure culturing vessels were constructed of ¾ inch 316 stainless steel tubing for 10 ml total capacity, and fitted with quarter turn plug valves (Swagelok or Hylok). Each column was loaded with 5 ml of medium containing appropriate amendments and endospores, prior to pressurization of the 5 ml remaining headspace to 10 MPa with CO 2 over a 1 h period. Cultures loaded in steel vessels were grown at 37 °C and shaking at 250 r.p.m. for 21 days prior to de-pressurization. The density of the scCO 2 phase under these conditions is 0.68 g ml –1 [70] . The pressure of each column was verified to ensure supercritical conditions were maintained throughout the experiment. 1 ml samples of cells were stained with Syto9 (Invitrogen) and filtered on 0.22 μm polycarbonate filters (Whatman) for cell visualization and enumeration by fluorescence microscopy [25] . The remaining cell culture was centrifuged at 21,000 × g for 5 min. For β-galactosidase production experiments, the cell pellets were retained and stored at –20 °C until analysis. For alcohol generation experiments, alcohols were extracted from the cell-free supernatant using ethyl acetate and an identical protocol to what was used for cultures grown under aerobic and 0.1 MPa CO 2 conditions. β-Galactosidase activity assays Cells from 0.1 MPa CO 2 and 10 MPa scCO 2 cultures were lysed by addition of 100 μl of Bacterial Protein Extraction Reagent (B-PER) (Thermo Scientific) to the previously collected cell pellets and vortexing for 30 min at room temperature. Soluble cellular protein was collected by centrifuging the lysed cell pellets for 20 min at 18,500 × g and 4 °C. Total protein content for each sample was determined using a Pierce BCA Protein Assay Kit (Thermo Scientific) according to the manufacture’s instructions, and measuring the resulting absorbance at 562 nm (Beckman DU600). To determine protein concentration, samples were compared to a standard curve generated using 0.05–1.0 mg ml –1 of bovine serum albumin (BSA) and the same protocol. B-PER negative control samples were also analyzed and subtracted from the total protein content of the lysed samples. To assay for β-galactosidase activity, lysed culture supernatant was added to assay buffer (0.1 M sodium phosphate buffer pH 8, 10 mM KCl, 1 mM MgSO 4 ) to a final volume of 800 μl in a plastic cuvette (VWR). Samples were equilibrated at room temperature prior to the addition of 200 μl of 4 mg ml –1 freshly prepared, β-galactosidase substrate o-nitrophenyl-β-D-galactoside (ONPG) (Sigma). Absorbance at 420 nm was collected every 15 s for 10 min using a Beckman DU600 spectrophotometer. The volume of lysed culture was adjusted to ensure the concentration of ONPG was not limiting during the assay. The initial rate of absorbance change was calculated for each sample and converted to μmol min –1 using 2130 M –1 cm –1 as the extinction coefficient for ONPG. Rates were normalized by total protein added to each reaction to generate a specific activity per unit total protein for each sample. Compound quantification Glucose, xylose, αKIV, and fermentation products (acetate, lactate, formate) were detected using an HPLC (Agilent 1200) with an Aminex HPX-87H anion exchange column (Bio-Rad). Cell-free supernatants were loaded onto the column with an inlet and outlet temperature of 35 °C and flow rate of 0.6 ml min –1 under isocratic conditions with 5 mM sulfuric acid. Compound concentrations were determined by integrating the refractive index detection chromatogram and comparison to a standard curve generated with known concentrations of each commercially available standard (Sigma). Purified standards were also used to determine retention times: glucose—9 min, xylose—9.7 min, αKIV—10.2 min, lactate— 13.0 min, formate—14.3 min, and acetate—15.6 min. Alcohols and isobutyraldehyde were detected using a gas chromatography system (Agilent 7890B GC) equipped with a VF-wax column (Agilent 30 m × 0.25 mm × 0.50 μm), flame-ionization detector (FID) and mass spectrometer (MS). All compounds were extracted into ethyl acetate from cell-free supernatants prior to analysis. The temperature program for the GC oven was 80 °C hold for 3 min, 5 °C min –1 ramp to 210 °C, and 210 °C hold for 3 min. Compound concentrations were determined by integrating the FID chromatogram and comparison to a standard curve generated with known concentrations of each commercially available standard (Sigma). To generate a standard curve using purified compounds, mixtures of compounds were extracted from LB or M9-based semi-defined medium using ethyl acetate, identical to the procedure for microbially generated compounds. Purified standards were also used to determine retention times, and identification of microbially produced compounds was confirmed using the MS fingerprint. The retention times for the molecules in this study are: isobutyraldehyde —4.2 min, isobutanol—7.2 min, isopentanol—8.9 min, and phenylethyl alcohol (PEA)—27.2 min. Yield of isobutanol on αKIV was calculated by dividing the moles of isobutanol produced by the moles of αKIV substrate consumed, noting a 1:1 molar relationship of aKIV conversion to isobutanol (Fig. 4a and Supplementary Table 4 ). To measure microbially generated compounds found in the scCO 2 headspace of high-pressure stainless steel columns, the headspace was de-pressurized directly into chilled ethyl acetate. The 316 stainless steel tubing and valves in a pressurization manifold [22] enabled the simultaneous de-pressurization of 12 samples. Compounds present in the ethyl acetate were analyzed by GC, as was performed for other extracted molecules. Prior to extraction, steel tubing was flushed with ethyl acetate to eliminate cross contamination. Isobutanol was also extracted from a custom built extractor-fermenter [12] using scCO 2 . A 1% w/v isobutanol (Sigma) solution was prepared in deionized water and extraction was carried out at scCO 2 flow rates of 1.3, 3.2, 5.4, and 9.0 ml min –1 . The scCO 2 was de-pressurized through chilled methanol to collect the isobutanol, which was quantified by GC-FID [12] . Recovery rate was determined by fitting the natural log of the fraction recovered as a function of time [12] . scCO 2 fermentation-extraction process model Aspen Plus (AspenTech) was used to simulate the isobutanol extraction process (full process: Supplementary Fig. 15a , simplified process schematic: Fig. 5a ). Preliminary calculations and comparison with published data [45] , [46] suggested use of the Soave-Redlich-Kwong equation of state to model phase equilibrium in all cases except for scCO 2 extraction of isobutanol, for which our own measurements on isobutanol were used in concert with literature data on n -butanol separation performance [43] , [44] . Thermodynamic properties were modeled using the Lee-Kessler-Plöcker equation of state, as recommended by Aspen for supercritical fluids. The process feeds were CO 2 at 0.1 MPa and a stream of aqueous glucose (media and substrate). The water feed (P1) was pumped to 10 MPa in a single stage. Consistent with typical engineering practice, CO 2 pressurization to 10 MPa was completed in four stages (C1-4), with each stage accomplishing a threefold pressure increase. In all cases, the thermodynamic efficiency of the pumps/compressors was 85% and their mechanical efficiency was 35%. Heat exchangers (HE1-3) were used to maintain CO 2 temperature at 40 °C after compression and for feeding the fermenter. The fermenter was simulated as consisting of a continuously fed stirred tank reactor and a separator (V2) configured in series. The reactor was modeled as achieving a steady state isobutanol concentration of 20 g l –1 , consistent with reported titers of isobutanol [27] . The entire contents of the reactor were fed to the separator (V2), a counter-current isobutanol extraction column [44] , which separated the feed into water-rich and CO 2 -rich streams. The isobutanol composition of the exit streams were set to that reported by Laitinen and Kaunisto [44] and modified using our performance data for isobutanol (i.e., 99.73% butanol recovery) and the exiting water and CO 2 streams were assumed to be at mutual saturation, using the data reported by King et al. [54] for binary mixtures. Downstream of the fermenter, a three-phase separator (V3) was used to decrease the pressure to permit the separation of isobutanol-rich, water-rich, and CO 2 -rich streams, as suggested by de Filippi and Moses [43] . Pressures tested in the three-phase separator ranged from 0.1 to 6.5 MPa, the pressure at which an isobutanol-rich phase first appears. The CO 2 -rich stream exiting the three-phase separator was either recycled or purged, with the ratio between these streams set by the splitter (V5). The CO 2 recycle ratio was defined by the relative mass flow rates of the CO 2 streams exiting the splitter; e.g., 50% CO 2 recycle implies that 50% of the CO 2 entering the splitter is recycled and 50% is off gassed. The isobutanol-rich phase was further de-pressurized to 0.1 MPa (V4), if necessary, to recover high-purity isobutanol liquid. Finally, the water exiting the three-phase separator was purged, though it could be recycled in an industrial process. Reporting Summary Further information on experimental design is available in the Nature Research Reporting Summary linked to this Article.